Abiotic ligation of DNA oligomers templated by their liquid crystal ordering It has been observed that concentrated solutions of short DNA oligomers develop liquid crystal ordering as the result of a hierarchically structured supramolecular self-assembly. In mixtures of oligomers with various degree of complementarity, liquid crystal microdomains are formed via the selective aggregation of those oligomers that have a sufficient degree of duplexing and propensity for physical polymerization. Here we show that such domains act as fluid and permeable microreactors in which the order-stabilized molecular contacts between duplex terminals serve as physical templates for their chemical ligation. In the presence of abiotic condensing agents, liquid crystal ordering markedly enhances ligation efficacy, thereby enhancing its own phase stability. The coupling between order-templated ligation and selectivity provided by supramolecular ordering enables an autocatalytic cycle favouring the growth of DNA chains, up to biologically relevant lengths, from few-base long oligomers. This finding suggests a novel scenario for the abiotic origin of nucleic acids. The experiments reported here were motivated by the recent demonstration of the liquid crystal (LC) ordering of ultrashort DNA and RNA oligomers in concentrated aqueous solutions [1] , [2] , resulting from the following steps of hierarchical self-assembly (HSA; sketched in Fig. 1a ); first, the pairing of sufficiently complementary oligomers into duplexes; second, the stacking of duplexes into linear aggregates via end-to-end attractive interactions, such as blunt-end base stacking, or the coupling of overhangs [3] , [4] ; third, the collective orientational ordering of the anisotropic aggregates; and finally, the discontinuous condensation, through phase separation, of LC droplet domains as the DNA concentration is increased to >400–500 g l −1 . The discontinuous onset of LC ordering requires this entire sequence of HSA steps, a multiplicative selection process that enables the LC domains to act effectively as gatekeepers, sequestering from the solution only those oligomers having a sufficient degree of complementarity and a sufficient tendency to end-to-end aggregation, while oligomers not meeting these requirements and other solute molecules not participating in the orientational ordering are physically expelled from the LC phase [4] , [5] . In addition to gathering sufficiently complementary molecules, the long-ranged LC orientational order greatly stabilizes end-to-end molecular contacts between these oligomers within the LC domains [6] , [7] , [8] , relative to those in the isotropic phase in which there are only transient interactions and short-ranged spatial correlations between neighbouring duplexes. 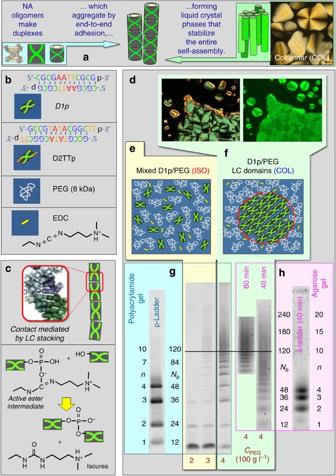Figure 1: Enhanced abiotic ligation afforded by the condensation of DNA into LC domains. (a) DNA oligomer duplexes having end-to-end attraction order into LC phases that in turn stabilize their linear aggregates. (b) Molecules used in this study are as follows: the self-complementary 12-mer D1p, the partially self-complementary 14-mer D2TTp, the flexible water-soluble polymer PEG (molecular weight=8,000) and the water-soluble carbodiimide EDC used as ligating agent. Both DNA oligomer have a 3′ phosphate terminus. The two sequences are chosen not to form mixed D1p/D2TTp duplexes. (c) Mechanisms of autocatalysis and ligation. LC-stabilized end-to-end interaction holds the 3′ phosphate and the 5′ hydroxyl terminals in physical contact. Inset is adopted from ref.8. EDC activates the phosphate terminal first, yielding an active intermediate that can react with the hydroxyl terminal to yield a native phosphodiester link, with isourea as by-product. (d) Phase behaviour and ligation in D1p/PEG/EDC/water mixtures. (e) At low PEG concentration, the mixture is a uniform isotropic solution. (f) ForcPEG>400 g l−1, the mixture phase separates into COL droplets of linearly aggregated duplexed DNA surrounded by an isotropic solution of PEG, as shown in the pictures above of the same 20-μm-thick flat cell in polarized and in fluorescence microscopy (duplexes are selectively marked by EvaGreen dye). (g) Fifteen per cent polyacrylamide gel stained by ethidium bromide. Three electrophoretic runs are shown as follows:cPEG=200 g l−1(uniform solution),cPEG=300 g l−1(few small COL domains) andcPEG=400 g l−1(COL domains). Correspondingly, the product distribution is greatly modified. (h) Agarose gel (3.5%) runs of thecPEG=400 g l−1sample recorded at two different run times. The picture of the 60-min run gel has been compressed and shifted to match the band position and spacing of the 40-min run gel, according to the band analysis described inSupplementary Methods. Numbers along the lanes indicate the oligomer lengths expressed in number of bases (Nb) and the polymerization number (n). In both gels, the ladder contains DNA oligomers 12, 24, 36 and 48 bases long, synthesized by repetition of D1p sequence. The straight line is a guide for the eyes marking the condition ofNb=120 (n=10). Full gel images are shown inSupplementary Figs 14 and 15. Figure 1: Enhanced abiotic ligation afforded by the condensation of DNA into LC domains. ( a ) DNA oligomer duplexes having end-to-end attraction order into LC phases that in turn stabilize their linear aggregates. ( b ) Molecules used in this study are as follows: the self-complementary 12-mer D1p, the partially self-complementary 14-mer D2TTp, the flexible water-soluble polymer PEG (molecular weight=8,000) and the water-soluble carbodiimide EDC used as ligating agent. Both DNA oligomer have a 3′ phosphate terminus. The two sequences are chosen not to form mixed D1p/D2TTp duplexes. ( c ) Mechanisms of autocatalysis and ligation. LC-stabilized end-to-end interaction holds the 3′ phosphate and the 5′ hydroxyl terminals in physical contact. Inset is adopted from ref. 8 . EDC activates the phosphate terminal first, yielding an active intermediate that can react with the hydroxyl terminal to yield a native phosphodiester link, with isourea as by-product. ( d ) Phase behaviour and ligation in D1p/PEG/EDC/water mixtures. ( e ) At low PEG concentration, the mixture is a uniform isotropic solution. ( f ) For c PEG >400 g l −1 , the mixture phase separates into COL droplets of linearly aggregated duplexed DNA surrounded by an isotropic solution of PEG, as shown in the pictures above of the same 20-μm-thick flat cell in polarized and in fluorescence microscopy (duplexes are selectively marked by EvaGreen dye). ( g ) Fifteen per cent polyacrylamide gel stained by ethidium bromide. Three electrophoretic runs are shown as follows: c PEG =200 g l −1 (uniform solution), c PEG =300 g l −1 (few small COL domains) and c PEG =400 g l −1 (COL domains). Correspondingly, the product distribution is greatly modified. ( h ) Agarose gel (3.5%) runs of the c PEG =400 g l −1 sample recorded at two different run times. The picture of the 60-min run gel has been compressed and shifted to match the band position and spacing of the 40-min run gel, according to the band analysis described in Supplementary Methods . Numbers along the lanes indicate the oligomer lengths expressed in number of bases ( N b ) and the polymerization number ( n ). In both gels, the ladder contains DNA oligomers 12, 24, 36 and 48 bases long, synthesized by repetition of D1p sequence. The straight line is a guide for the eyes marking the condition of N b =120 ( n =10). Full gel images are shown in Supplementary Figs 14 and 15 . Full size image Here we show that, with the addition of the appropriate chemistry, this unique combination of selectivity, molecular arrangement and fluidity provided by the LC ordering strongly promotes the covalent coupling of the oligomers of neighbouring stacked duplexes into longer complementary strands. Such polymerization, in turn, generically stabilizes LC order, enhancing it in a positive feedback system of HSA, selection and synthesis, which we describe as LC autocatalysis, and propose as a path towards the abiotic appearance of self-assembling liner polymers. Description of ligation strategy Abiotic ligation experiments are carried out in aqueous solutions containing DNA oligomers and the water-soluble ligating agent 1-ethyl-3-(3-dimethylaminopropyl) carbodiimide (EDC; Fig. 1b and ref. 9 ). EDC activates the phosphate terminals, so that they can react with hydroxyl terminals to generate a native covalent phosphodiester bond, with isourea as a by-product as sketched in Fig. 1c (details in Supplementary Note 1 and Supplementary Fig. 1 ). We investigate ligation in solutions of EDC and the self-complementary Dickerson dodecamer 3′ phosphate (5′- CGCGAATTCGCGp -3′, D1p), shown in extensive previous study to organize into isotropic (ISO), nematic (NEM) or columnar (COL) LC phases [1] , depending on concentration and temperature T . EDC-activated phosphate terminals can also react with water, in this case producing isourea and a phosphate terminal ready to react again with another EDC molecule ( Supplementary Note 2 ). We observe that the solubility of EDC in the LC phases is limited to molar ratios R =[EDC]/[D1p]<3, a condition that does not allow an EDC supply large enough to generate significant polymerization. This limitation is effectively bypassed by exploiting the self-selection properties of phase separation. We thus dilute DNA by a solution of polyethylene glycol (PEG), a chemically inert water-soluble polymer often used as a depletant to control osmotic pressure Π (refs 10 , 11 ). Previous experiments [5] indicated that as the PEG concentration ( c PEG ) is providing a large enough Π , the solution phase separates into DNA-rich COL LC domains surrounded by a PEG-rich isotropic fluid ( Fig. 1f ). Therefore, DNA solutions with a concentration c DNA much smaller than c DNALC , which is necessary to induce LC ordering in a pure water–D1p solution, are homogeneously mixed with PEG at low c PEG ( Fig. 1e ), but for sufficiently large c PEG , D1p LC COL domains will appear, surrounded by an isotropic phase that contains EDC at values of R that can be orders of magnitude larger than above, typically in the range 10< R <50. The properties of the LC condensate depend only on Π , which in this case is mainly provided by PEG and to a lesser extent by EDC and isourea, but could, in principle, be provided by single-stranded DNA or by ill-terminating duplexes [4] , [5] . In these conditions, and by virtue of the intrinsic self-selection properties of phase separation [12] , LC domains, constituting only a small fraction of the entire sample volume, act as microreactors having a state established by T and Π , effective access to reactants, and a large waste sink. Samples are prepared by dissolving a small amount of lyophilized D1p in fresh prepared EDC mixture with PEG at various c PEG =100–400 g l −1 to obtain a homogeneous solution with c DNA ~0.05 c DNALC and R =50. Experiments are carried out in parallel in small plastic tubes and in flat cells to enable visual confirmation of LC domains formation through light microscopy. Tests revealed that the ligation reaction was completed in ~24 h, so we set this as the incubation time for all the experiments reported here, terminating the reaction at the end by 20-fold dilution with 50 mM ethanolamine (details in Methods section). Enhanced ligation in LC domains segregated from PEG Typical 15% polyacrylamide gel scans of DNA extracted from such solutions are shown in Fig. 1g , where the signal is given by the fluorescent emission provided by ethidium bromide staining (details in Supplementary Methods ). Ligation in the low c PEG homogeneous mixtures is limited even at this relatively high c EDC , but the appearance of condensed droplets with LC ordering produces a qualitatively new behaviour, manifested by the growth of a large peak in oligomer population having a mean degree of polymerization, ‹ n ›>10. To better visualize the length distribution, the same samples are also run in 3.5% agarose gels where the bands associated with longer oligomers are more easily distinguished ( Fig. 1h ). Profiles of the fluorescent emissions of the gel runs are presented in Fig. 2 and analysed by exploiting the approximate proportionality between electrophoretic mobility and logarithm of chain length [13] (details in Supplementary Methods and Supplementary Figs 2–4 ). Despite the intrinsic uncertainty in the quantitative information carried by the fluorescence profiles of the gels, the product length distribution P(n) extracted from the profiles is well described by a simple Flory model [14] ( Supplementary Note 3 , Supplementary Methods and Supplementary Figs 5–7 ). This enables quantification of the increment in polymerization yield (Flory parameter, p ) owing to the phase separation and LC condensation: from p ~0.13 ( c PEG =200 g l −1 , mixed D1p/PEG ISO phase) to p ~0.84 ( c PEG =400 g l −1 , D1p LC COL domains), as shown in Fig. 2a for the polyacrylamide gel runs. Moreover, integration of the agarose gel profile in Fig. 2b indicates that in the COL domains 20% (10%) of the DNA mass is part of chains with n >30 ( n >50) and that ‹ n ›~19, corresponding to oligomers of N b =12 n =208 base pairs. 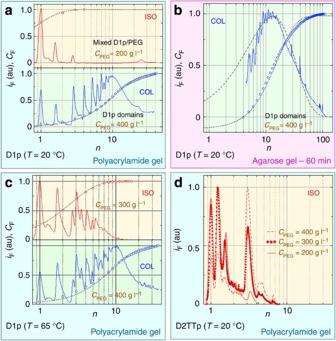Figure 2: Fluorescence intensity profiles of the gel electrophoresis runs. Measurements are performed on DNA/PEG/EDC mixtures, and gels are stained by ethidium bromide. Plots are shown as a function ofn, the position along the gel converted in degree of polymerization (Supplementary Methods).iF(n)(continuous lines) is the fluorescence intensity.CF(n)(open dots) is the cumulative weight fraction distribution, obtained integratingiF(n)(Supplementary Methods). Dotted lines ina–cand the dashed line inbhave been obtained by fitting the data with the Flory model for simple polymerization from which the polymerization yieldphas been determined (seeSupplementary Figs 6 and 7). Dotted lines:C(n),Supplementary Equation (3). Dashed line:P(n),Supplementary Equation (2). (a) D1p/PEG/EDC mixtures measured in a 15% polyacrylamide gel for increasing PEG concentration:cPEG=200 g l−1, red lines (upper panel), uniform isotropic DNA/PEG/EDC mixture, ‹n›<2,p≈0.13;cPEG=400 g l−1, blue lines (lower panel), DNA COL domains in a PEG ISO background, ‹n›≈11,p≈0.84. ThecPEG=300 g l−1profile (not shown) can be obtained by a superposition of thecPEG=200 g l−1andcPEG=400 g l−1profiles, consistent with the appearance of a few small DNA COL domains. (b) D1p/PEG/EDC mixtures forcPEG=400 g l−1measured in 3.5% agarose gels for 60 min running time. At this long running time, enabling better detection of longer products, the first detectable peak corresponds ton=5. Analysis indicates ‹n›≈19 andp≈0.90. (c) D1p/PEG/EDC mixtures measured atT=65 °C. Upper panel:cPEG=300 g l−1, D1p-rich ISO phase coexisting with a PEG-rich ISO phase, ‹n›≈3.5,p≈0.49. Lower panel:cPEG=400 g l−1, D1p-rich COL domains coexisting with a PEG-rich ISO phase, ‹n›≈10,p≈0.81. (d) D2pTT/PEG/EDC mixtures at variouscPEG, yielding uniform mixtures (cPEG=200) or condensation of COL domains (cPEG≥300 g l−1; ‹n›<3. Figure 2: Fluorescence intensity profiles of the gel electrophoresis runs. Measurements are performed on DNA/PEG/EDC mixtures, and gels are stained by ethidium bromide. Plots are shown as a function of n , the position along the gel converted in degree of polymerization ( Supplementary Methods ). i F (n) (continuous lines) is the fluorescence intensity. C F (n) (open dots) is the cumulative weight fraction distribution, obtained integrating i F (n) ( Supplementary Methods ). Dotted lines in a – c and the dashed line in b have been obtained by fitting the data with the Flory model for simple polymerization from which the polymerization yield p has been determined (see Supplementary Figs 6 and 7 ). Dotted lines: C ( n ), Supplementary Equation (3) . Dashed line: P ( n ), Supplementary Equation (2) . ( a ) D1p/PEG/EDC mixtures measured in a 15% polyacrylamide gel for increasing PEG concentration: c PEG =200 g l −1 , red lines (upper panel), uniform isotropic DNA/PEG/EDC mixture, ‹ n ›<2, p ≈0.13; c PEG =400 g l −1 , blue lines (lower panel), DNA COL domains in a PEG ISO background, ‹ n ›≈11, p ≈0.84. The c PEG =300 g l −1 profile (not shown) can be obtained by a superposition of the c PEG =200 g l −1 and c PEG =400 g l −1 profiles, consistent with the appearance of a few small DNA COL domains. ( b ) D1p/PEG/EDC mixtures for c PEG =400 g l −1 measured in 3.5% agarose gels for 60 min running time. At this long running time, enabling better detection of longer products, the first detectable peak corresponds to n =5. Analysis indicates ‹ n ›≈19 and p ≈0.90. ( c ) D1p/PEG/EDC mixtures measured at T =65 °C. Upper panel: c PEG =300 g l −1 , D1p-rich ISO phase coexisting with a PEG-rich ISO phase, ‹ n ›≈3.5, p ≈0.49. Lower panel: c PEG =400 g l −1 , D1p-rich COL domains coexisting with a PEG-rich ISO phase, ‹ n ›≈10, p ≈0.81. ( d ) D2pTT/PEG/EDC mixtures at various c PEG , yielding uniform mixtures ( c PEG =200) or condensation of COL domains ( c PEG ≥300 g l −1 ; ‹ n ›<3. Full size image These results show that the chemical ligation of DNA oligomers into linear chains is greatly enhanced by COL ordering. Mechanisms contributing to this enhancement include the organization of the duplexes into the base pair stacks characteristic of the already ligated bases; the promotion of the ligation reaction by maintenance of continuous stable proximity (high local concentration) of the reacting terminals, according to the law of mass action; the provision by the LC phase of a fluid environment for transport and reaction, and the coexistence of phases that provides an ISO environment surrounding the LC domains in which EDC can freely diffuse. In this way, the limitations of the finite solubility of EDC in the COL phase are overcome by a continuous supply from the ISO phase. Gel data from ligation in the COL phase ( Fig. 1d ) show a very strong depletion of the monomer band, indicating that such EDC supply mechanism combined with the reaction time (~1 day; Supplementary Note 4 and Supplementary Fig. 8 ) ensure that the largest part of the duplexes within the COL domains takes part in the reaction. Comparison of ligation in ISO and LC phases To discriminate the individual relevance of DNA LC ordering versus the local increase in c DNA provided by phase separation, we exploit the new observation that PEG can phase separate droplets of concentrated duplexed DNA oligomers in either the ISO or the LC COL phase, depending on T , c PEG and oligomer structure. This provides us the opportunity to compare ligation efficiencies between conditions where the only significant difference is the LC ordering, which is pursued in two distinct experiments. In a first experiment, we compare ligation of D1p in ISO and COL at the same T and different Π . Indeed, we find that at T ~65 °C, a T at which the COL phase melts but D1p duplexes are still stable, condensation of D1p into the ISO phase is possible (details in Methods section and Supplementary Figs 9 and 10 ). This behaviour contrasts the one observed at T =20 °C, where, upon increasing c PEG , D1p condenses directly into the COL phase. Specifically, by maintaining a constant T =65 °C, we select and study in parallel the ligation of D1p at c PEG =300 g l −1 , at which the DNA phase separates from PEG into ISO droplets ( Fig. 3b ), and at c PEG =400 g l −1 , where COL domains are found ( Fig. 3c ). Optical observation and simulated phase diagram versus Π (ref. 6 ) indicate that c DNA is very similar in these two condensed phases, being no >10% larger in the COL. The data of the resulting gel runs are shown in Fig. 3e , with the intensity profile plotted in Fig. 2c . The difference in the product length distribution directly attributable to the LC ordering is quite marked, analysis of the curves yielding ‹ n ›≈3.5 in the ISO phase and ‹ n ›≈10 in the COL phase (details in Supplementary Note 5, 6 and Supplementary Figs 11–13 ). 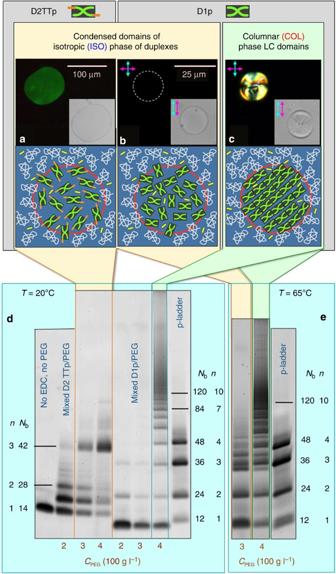Figure 3: Ligation in condensed LC and isotropic DNA droplets. (a) Sketch, bright-field and fluorescent emission microscope picture of condensed D2TTp ISO droplets in a D2TTp/PEG mixture atT=20 °C. Duplexes are selectively marked by EvaGreen dye. (b) Sketch and polarized microscope images (crossed and parallel polarizers) of ISO D1p droplets in a D1p/PEG/EDC mixture atT=65 °C andcPEG=300 g l−1, respectively. (c) Sketch and polarized microscope images (crossed and parallel polarizers) of COL D1p droplets in a D1p/PEG/EDC mixture atT=65 °C andcPEG=400 g l−1, respectively (identical structures are found at 20 °C). (d) Polyacrylamide gel (15%) comparing the ligation products in D1p and D2TTp in identical conditions. The formation of concentrated DNA domains produces in the case of D2TTp (lanes on the left-hand side of the gel) a minor increment in the product length, contrasting with the marked discontinuity in the case of D1p. (e) Polyacrylamide gel (15%) comparing the ligation products obtained in D1p/PEG/EDC atT=65 °C, where, depending oncPEG, the system is either uniformly mixed or it partitions into two coexisting ISO phases (cPEG=300 g l−1, sketchb), or else it phase separates into coexisting COL and ISO phases (cPEG=400 g l−1, sketchc). Numbers along the lanes indicate the oligomer lengths expressed in number of bases (Nb) and the polymerization number (n). In both gels, the ladder contains DNA oligomers 12, 24, 36 and 48 bases long, synthesized by repetition of D1p sequence. The straight lines are a guide for the eyes, helping the identification of bands corresponding to selectedNb. Full gel images are shown inSupplementary Fig. 16. Figure 3: Ligation in condensed LC and isotropic DNA droplets. ( a ) Sketch, bright-field and fluorescent emission microscope picture of condensed D2TTp ISO droplets in a D2TTp/PEG mixture at T =20 °C. Duplexes are selectively marked by EvaGreen dye. ( b ) Sketch and polarized microscope images (crossed and parallel polarizers) of ISO D1p droplets in a D1p/PEG/EDC mixture at T =65 °C and c PEG =300 g l −1 , respectively. ( c ) Sketch and polarized microscope images (crossed and parallel polarizers) of COL D1p droplets in a D1p/PEG/EDC mixture at T =65 °C and c PEG =400 g l −1 , respectively (identical structures are found at 20 °C). ( d ) Polyacrylamide gel (15%) comparing the ligation products in D1p and D2TTp in identical conditions. The formation of concentrated DNA domains produces in the case of D2TTp (lanes on the left-hand side of the gel) a minor increment in the product length, contrasting with the marked discontinuity in the case of D1p. ( e ) Polyacrylamide gel (15%) comparing the ligation products obtained in D1p/PEG/EDC at T =65 °C, where, depending on c PEG , the system is either uniformly mixed or it partitions into two coexisting ISO phases ( c PEG =300 g l −1 , sketch b ), or else it phase separates into coexisting COL and ISO phases ( c PEG =400 g l −1 , sketch c ). Numbers along the lanes indicate the oligomer lengths expressed in number of bases ( N b ) and the polymerization number ( n ). In both gels, the ladder contains DNA oligomers 12, 24, 36 and 48 bases long, synthesized by repetition of D1p sequence. The straight lines are a guide for the eyes, helping the identification of bands corresponding to selected N b . Full gel images are shown in Supplementary Fig. 16 . Full size image In a second experiment, we compare ligation at T =20 °C and equal Π in the PEG-induced condensed phases of two different DNA sequences: D1p and 5′- GCCGTATACGGC TTp -3′ (D2TTp). D2TTp is a self-complementary dodecamer sequence (underlined section) with two additional T bases on the 3′ end. Hence, D2TTp forms duplexes terminating in non-pairing TT overhangs that suppress end-to-end duplex adhesion and thus LC ordering. We thus explore PEG/D2TT/EDC mixtures ( R =50, variable c PEG ) according to the protocol described above and characterize the products by gel electrophoresis. We find phase separation of ISO droplets ( Fig. 3a ) for c PEG >300 g l −1 . The condensation of DNA-rich ISO droplets of D2TTp brings about a much smaller effect in the ligation efficiency than the condensation of the D1p LC droplets, as visible in the gel runs ( Fig. 3d ) and in their intensity profiles ( Fig. 2d ). The appearance of bands in the gel not corresponding to multiple of D2TTp, probably indicating the formation of circular products, makes impossible the semi-quantitative analysis with the Flory model used above. However, the intensity profiles can be directly integrated to extract ‹ n ›, which yields ‹ n ›<3 even at the largest c PEG . These results clearly support the notion that phase separation and LC ordering are both essential factors in the self-assembly-induced enhancement of the abiotic EDC-based ligation used here. LC ordering provides continuous close contact between the reacting terminals, without which no significant elongation is observed. However, phase separation is crucial as well; it selectively confines the DNA LC into domains whose internal fluid structure bounded by an aqueous/aqueous interface that enables easy transport of material, proving to be a convenient and effective arrangement to carry out the ligation reaction. Selectivity of LCs microreactors It is clear from these and earlier experiments that in a mixture of oligomers, the selectivity afforded by the cascaded phase separation of sequences provides an effective self-sorting mechanism by rejecting, for example, the entry of single strands into the LC domains [1] , [5] , or else admitting duplexes with sufficiently adhesive tails, such as in solutions of complementary duplexes with overhangs [3] or of random sequence DNA oligomers [4] . In systems such as oligomeric DNA, where the modes of self-assembly are strongly interdependent, sequence dependent and hierarchical (for example, end-to-end adhesion of oligomers is more or less irrelevant if they are not duplexed), phase separation also becomes a type of staged or cascaded selection mechanism, manifested in a cascade of thermodynamic instabilities. This is illustrated in Fig. 4 (for a more detailed discussion, see Supplementary Note 7 and Supplementary Table 1 ), displaying the phase coexistence observed in a three-component mixed solution of D1p, D2TTp and PEG. At low PEG concentration, these solutions are single phase, consisting of random coil PEG and duplexed DNA oligomers. For c PEG >300 g l −1 , the DNA duplexes phase separate from PEG, a result of their compact rigid structure, originating in their hybridized portions. As the concentration of duplexed DNA locally increases because of this PEG versus DNA phase separation, a second-phase separation takes place between the isotropic (ISO) and columnar (COL) LC phases, the COL phase principally comprises blunt-end D1p and the ISO phase is mainly composed of D2TTp, which cannot form LCs. Thus, this second-phase separation is carried in a context that is created by the first. These staged partitioning acts as a hierarchical selection mechanism, condensing together the blunt-ended D1p duplexes that enable LC ordering, which are precisely those in which contacting terminals promote enhanced ligation. 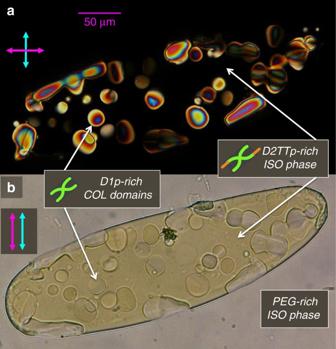Figure 4: Three-phase coexistence in a D1p/D2TTp/PEG mixture. Optical microscopy images of 20-μm-thick flat cell containing a D1p/D2TTp/PEG mixture with [D1p]/[D2TTp]≈1 andcPEG=300 g l−1. The same cell is imaged through crossed (a) and parallel (b) polarizers. Coloured COL domains are visible ina. The internal alignment of the COL domains is nearly uniform, the colours depending mainly on the domain thickness. (b) The coexistence of three phases are as follows: the DNA COL domains, the DNA ISO phase (black inaand pale yellow inb) and the PEG-rich ISO phase background (details inSupplementary Note 7). Figure 4: Three-phase coexistence in a D1p/D2TTp/PEG mixture. Optical microscopy images of 20-μm-thick flat cell containing a D1p/D2TTp/PEG mixture with [D1p]/[D2TTp]≈1 and c PEG =300 g l −1 . The same cell is imaged through crossed ( a ) and parallel ( b ) polarizers. Coloured COL domains are visible in a . The internal alignment of the COL domains is nearly uniform, the colours depending mainly on the domain thickness. ( b ) The coexistence of three phases are as follows: the DNA COL domains, the DNA ISO phase (black in a and pale yellow in b ) and the PEG-rich ISO phase background (details in Supplementary Note 7 ). Full size image In the formulation of origin-of-life scenarios, self-assembly is often invoked [15] , [16] as the only available mechanism to bridge the ‘insurmountable kinetic barrier’ [17] connecting simple carbon-based molecules available on the early Earth and the simplest structures capable of enzymatic activity [18] , which in a RNA world scenario would be ribozymes [19] , [20] . Here we have offered a real example, based on DNA but very likely extendable to RNA [3] or other nucleic acid precursors [21] , of how this path could have actually taken place, showing that the interplay of fluid ordering, aqueous phase separation, and distinctive modes of hierarchical and sequence-directed self-assembly can direct chemical reaction in a way that facilitates production of long chains of variable sequence. We envision our findings as a paradigm of what could have happened in the prebiotic Earth based on the fundamental and simplifying assumption that the origin of nucleic acids is written in their structure. This vision combines well with the classic notions of thermal and drying–wetting cycles, generally considered basic drivers for life to emerge on early Earth [22] , [23] , and with more recent notions such as the thermophoretic accumulation of DNA-like molecules in hydrothermal pore systems [24] , [25] , thereby offering a plausible pathway for the molecular crowding crucial for LC ordering to appear. Future research will have to focus on what could have preceded the processes outlined here—clarifying the minimal ingredients that enable condensation of DNA LC domains in complex molecular environments, and what could have followed it—determining the first crucial enzymatic activities enhancing and maybe guiding the LC-assisted ligation towards an elementary form of (pre)biological evolution. Materials The materials used in this study are as follows: 5′-hydroxy-3′-phosphate deoxyribonucleotide oligomers 12-mer D1p, 5′-OH- CGCGAATTCGCG -p-3′, and 14-mer D2TTp, 5′-OH- GCCGTATACGGCTT -p-3′, HPLC purity grade (Primm); 4-(2-hydroxyethyl)-1-piperazineethanesulfonic acid and HEPES buffer (Sigma); water-soluble EDC (Sigma) and PEG, molecular weight=8 kDa (Fluka). Samples preparation and reactions Reactions are performed in glass thin flat cells of 20 μm width (to be observed at the microscope—1 μl total reaction volume) and in Eppendorf plastic tubes (2–10 μl total reaction volume). In both cases, samples are prepared by solubilizing lyophilized DNA by aqueous PEG/EDC solutions in 0.01 M HEPES buffer (pH 7.55). Amounts are chosen to obtain a concentration of oligomers c 0 =5 mM and a PEG concentration variable in the range c PEG =100–400 g l −1 . Solutions are prepared with freshly hydrated EDC, with EDC/DNA molar ratios R =50. Both thin flat cells and tubes are sealed by oil to prevent evaporation. Reaction temperature is 25 °C (controlled by Instec hot stage), with the exception of the experiments in which LC melting is induced by rising the temperature to 65 °C. After 24 h from the preparation of the solutions, reactions are stopped by 20-fold dilution in 50 mM ethanolamine (Sigma). Observation of LC phases Cells are observed with either a Nikon TE200 or a Nikon Optiphot2 polarized microscopes and images are acquired on Nikon DS-5M and Prosilica GX-1050 b/w CCD cameras. Fluorescent images are obtained by doping DNA with EvaGreen dye (Biotium). The optical properties of LC phases directly reflect the symmetry of their ordering. Birefringence, the anisotropy of the refractive index, is determined by the quality of the local collective molecular orientation. Simple inspection of LC samples in thin cells by polarized transmission light microscopy enables detecting the presence of LC phases, which will appear coloured, while the light transmitted by isotropic liquids, such as PEG solution, is extinguished by crossed polarizers. Moreover, the features of the optical textures associated to LC domains (type of deformation, domain boundaries and topological defect lines) generally enable determining the specific kind of LC phase. In the circumstances of this study, where the need is to distinguish isotropic, nematic and columnar phases—the only LC phases observed in DNA solutions, microscope observations are thus enough to characterize the samples. Melting of LC phase The LC domains melt as T is raised. The melting of the columnar LC phase has been characterized by observing the disappearance of birefringent LC textures upon increasing T as controlled by a microscope hot and cold stage (Instec HCS301i). Previous observations indicated that the melting of the LC phases of the Dickerson dodecamer takes place at a lower temperature than the one for the duplex melting (that is, the unbinding of the two strands) by 3–15 °C depending on concentration and ionic strength [3] , [4] . In mixtures of D1p and PEG, we observe dependence of the LC melting temperature on the PEG concentration. This is expected since a larger PEG concentration corresponds to higher osmotic pressure and larger DNA concentration inside the LC domains. Example of LC melting in D1p/PEG mixtures at c PEG =400 g l −1 is shown in Supplementary Fig. 9 . Crucial in the context of this work is the fact that at T>T MELT the DNA-rich domains remain separated from PEG-rich phase. This behaviour, in conjunction with the D1p/PEG phase behaviour described in the next paragraph, allowed us to compare ligation in isotropic versus LC DNA domains at similar DNA concentrations at T =65 °C and with different PEG concentrations. Phase diagram of D1p/PEG mixtures The phase diagram of mixtures of D1p, at fixed concentration c D1p =5 mM≈19 mg ml −1 , and PEG 8 kDa has been extensively investigated in function of c PEG and T . The following two regimes are found: at low c PEG the system shows a uniform phase of mixed D1p and PEG, whereas at high enough c PEG D1p-rich LC domains nucleate and coexist with the isotropic PEG-rich phase. Isotropic DNA-rich domains segregated from PEG are not found at room temperature, but are instead observed at higher T ( Supplementary Fig. 10 ). This behaviour indicates that at room T , the PEG-provided osmotic pressure needed to induce D1p/PEG phase separation is larger than the osmotic pressure at which the LC ordering of D1p sets in. At higher T , the two threshold values of osmotic pressure invert, enabling liquid–liquid phase coexistence. This behaviour will be the object of further studies. Concentration measurements DNA concentration in sealed flat cells is measured by microscope-based interferometry; details in Supplementary Methods . DNA concentration in diluted stock solutions is measured with NanoDrop 2000 (Thermo Scientific). Polyacrylamide gel electrophoresis A vertical polyacrylamide gel electrophoresis setup (Bio-Rad Protean II) is used for oligomers size separation. An amount of 5 μg of previously dried DNA are rehydrated with 10 μl of formamide and 3 μl of gel loading solution (30% glycerol, 0.025% bromophenol blue, 0.25% xylene cyanol and water), and loaded in denaturing polyacrylamide gel (0.75–1.5 mm thick, 7 M urea, TBE buffer and acrylamide:bisacrylamide 37.5:1), and run for 1–4 h at 30 V cm −1 voltage. Gels are stained for 20 min in 0.5 μg ml −1 EtBr TBE buffer, viewed on ultraviolet–visible transilluminator and images are acquired with Typhoon-9200 Phosphor Imager (Amersham Pharmacia Biotech). The ladder is the same for each gel and it is composed of DNA oligomers synthesized with repetitions of the D1p 12-mer sequence (12-mer 5′- CGCGAATTCGCG -3′, 24-mer 5′- CGCGAATTCGCGC - GCGAATTCGCG -3′, 36-mer 5′- CGCGAATTCGCG - CGCGAATTCGCG - CGCGAATTCGCG -3′ and 48-mer 5′- CGCGAATTCGCG - CGCGAATTCGCG - CGCGAATTCGCG - CGCGAATTCGCG -3′ from Biomers). Details in Supplementary Methods . Gels intensity profiles analysis Grey scale 16-bit images of the gels are processed with MacBiophotonics ImageJ software. Some gel images in the main text are cropped, in order to facilitate visualization, full gel images are shown in Supplementary Figs 14–16 . Quantitative comparison between samples are made for lanes belonging to the same gel. The fluorescence intensity profile of each lane is extracted by averaging on rectangular areas covering the full width of the gel lane. Optimal range of electrophoretic separation and signal linearity are discussed in Supplementary Methods and Supplementary Figs 2–4 . The intensity profile analysis is performed with a MATLAB code (details in Supplementary Methods and Supplementary Figs 6 and 7 ). How to cite this article: Fraccia, T. P. et al . Abiotic ligation of DNA oligomers templated by their liquid crystal ordering. Nat. Commun. 6:6424 doi: 10.1038/ncomms7424 (2015).